FAT10 and NUB1L bind to the VWA domain of Rpn10 and Rpn1 to enable proteasome-mediated proteolysis FAT10 is the only ubiquitin-like modifier that can target proteins for degradation by the proteasome in a ubiquitin-independent manner. The degradation of FAT10-linked proteins by the proteasome is strongly accelerated by the ubiquitin-like–ubiquitin-associated protein NEDD8 ultimate buster-1 long (NUB1L). Here we show how FAT10 and NUB1L dock with the 26S proteasome to initiate proteolysis. We identify the 26S proteasome subunit hRpn10/S5a as the receptor for FAT10, whereas NUB1L can bind to both Rpn10 and Rpn1/S2. Unexpectedly, FAT10 and NUB1L both interact with hRpn10 via the VWA domain. FAT10 degradation in yeast shows that human Rpn10 can functionally reconstitute Rpn10-deficient yeast and that the VWA domain of hRpn10 suffices to enable FAT10 degradation. Depletion of hRpn10 causes an accumulation of FAT10-conjugates also in human cells. In conclusion, we identify the VWA domain of hRpn10 as a receptor for ubiquitin-like proteins within the 26S proteasome and elucidate how FAT10 mediates efficient proteolysis by the proteasome. A central proteolytic pathway in eukaryotic cells is the ubiquitin–proteasome system [1] . The 26S proteasome is a complex of 2.5 MDa comprising the 19S regulatory particle (RP, also called PA700) and a 20S cylindrical core particle (CP). The RP is required for the binding and unfolding of poly-ubiquitylated proteins to enable their degradation. The RP can be subdivided into a base composed of six ATPases (Rpt 1–6) and four non-ATPases Rpn2/S1, Rpn1/S2, Rpn13, and Rpn10 and a lid composed of nine structurally diverse subunits. The major known ubiquitin receptors on the proteasome are the RP subunits Rpn10 (designated hRpn10 or S5a in humans [2] , [3] ) and Rpn13 (Adrm1 in humans [4] ) while the ATPase subunit Rpt5/S6′ has been cross-linked to poly-ubiquitin chains but evidence for its functional involvement in proteolysis is lacking [5] . Rpn10 is assumed to lie at the interface of the lid and the base [6] . This subunit comprises the N-terminal von Willebrand A (VWA) domain [7] and C-terminal ubiquitin interacting motifs (UIM1 and UIM2, together referred as UIMs) [8] , [9] , [10] . Polyubiquitin chains which are covalently attached to the lysine of substrates interact with Rpn10 via the ubiquitin interacting motifs (UIMs) [11] , [12] , [13] and with Rpn13 via the pleckstrin-like receptor for ubiquitin (Pru) domain [4] , [14] . In addition, there are further receptors for ubiquitin conjugates belonging to the ubiquitin-like–ubiquitin-associated (UBL–UBA) family of proteins, such as Rad23, Dsk2, and Ddi1, which only temporarily associate with the proteasome [15] . This indirect pathway involves interaction of ubiquitin chains with their carboxy-terminal UBA domains whereas their amino-terminal UBL domains interact with the Rpn1, Rpn2 or Rpn10 subunits of the proteasome [16] , [17] , [18] , [19] . FAT10 (HLA-F locus adjacent transcript 10) is an 18-kDa protein that has two ubiquitin-like domains with an identity of 29 and 36% to ubiquitin in its N- and C-terminal parts, respectively [20] . Several ubiquitin-like modifiers have been described but FAT10 is the only one that functions similarly to poly-ubiquitin as a tag for proteasome targeting [21] , [22] , [23] . The expression of FAT10 is strongly and synergistically induced in the presence of the proinflammatory cytokines interferon gamma (IFN-γ) and tumour necrosis factor alpha (TNF-α) [24] , [25] . Cytokine-treated cells show an extensive high-molecular-weight smear of FAT10 conjugates reminiscent of ubiquitin conjugates, and proteasome inhibition leads to the accumulation of FAT10 conjugates [23] , [26] , [27] . The E1 and E2 enzymes that mediate FAT10 conjugation have recently been identified as UBA6 and USE1, respectively [23] , [26] , [28] , [29] , [30] . The degradation of FAT10 and FAT10 conjugates is strongly accelerated by the scaffold protein NEDD8 ultimate buster-1 long (NUB1L), which is induced by interferons and contains a N-terminal UBL domain and three C-terminal UBA domains [22] , [31] , [32] . NUB1L binds to FAT10 via its 3 UBA domains and the 26S proteasome via hRpn10 (ref. 33 ). NUB1L may hence serve as a linker between FAT10 and the proteasome. However, FAT10 can also bind directly to the proteasome, and the deletion of the UBA domains of NUB1L interferes with FAT10 binding but not with the acceleration of FAT10 degradation [34] . The latter effect requires the UBL domain of NUB1L, which is needed for binding to the proteasome, suggesting a 'facilitator' function of NUB1L in FAT10-mediated degradation, reminiscent of the function of the Rpn10 VWA domain in Rad23-mediated degradation of poly-ubiquitylated substrates [19] . In this study, we aimed to elucidate the mechanism of accelerated degradation of FAT10 by NUB1L by identifying the interacting subunits of the 26S proteasome for FAT10 and NUB1L and by characterizing their function for FAT10-dependent degradation. We show that FAT10 docked to hRpn10 and NUB1L to hRpn10 or hRpn1. Both FAT10 and NUB1L bound to the VWA domain of Rpn10 that sufficed to reconstitute FAT10 degradation in yeast. Therefore, the VWA domain of Rpn10 serves as a receptor domain for UBL proteins at the 26S proteasome that mediates FAT10-dependent degradation. 19S RP subunits interacting with FAT10 and NUB1L To identify the subunit(s) within the 19S RP that mediate FAT10 and NUB1L binding to the proteasome, interaction of each individual 19S RP subunit with FAT10 and NUB1L was analysed in a yeast two-hybrid assay. hRpn10 was the only subunit for which an interaction with FAT10 could be detected ( Fig. 1a ). hRpn10 also interacted with NUB1L ( Fig. 1b ), confirming this previously described interaction [33] . The previously established interaction of FAT10 with NUB1L was used as a positive control [32] . Taken together, these results suggest that FAT10 and NUB1L binding to the proteasome occurs via a common 19S RP subunit, hRpn10. 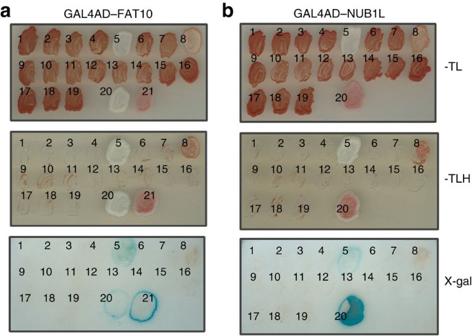Figure 1: hRpn10 interacts with FAT10 and NUB1L in a yeast two-hybrid assay. (a) Yeast two-hybrid analysis of the interaction of FAT10 with individual subunits of the human 19S RP. AH109 cells were co-transformed with pGADT7–FAT10 and a pGBD vector encoding one of the human 19S RP subunits fused to GAL4-BD. The colonies represent co-transformants with pGADT7–FAT10 and the indicated pGBD construct: (1) S1/Rpn2, (2) S2/Rpn1, (3) S3/Rpn3, (4) S4/Rpt2, (5) S5a/Rpn10, (6) S5b, (7) S6a/Rpt5, (8) S6b/Rpt3, (9) S7/Rpt1, (10) S8/Rpt6, (11) S9/Rpn6, (12) S10a/Rpn7, (13) S10b/Rpt4, (14) S11/Rpn9, (15) S12/Rpn8, (16) S13/Rpn11, (17) S14/Rpn12, (18) S15, (19) p55/Rpn5. (20) As positive control, we co-transformed the NMY51 cells with pGADT7–NUB1L and pLexA–FAT10. A second positive control (21) was the known interaction of NUB1L and hRpn10. Transformants were grown on selection plates containing 3-AT but lacking tryptophan and leucine (−TL) or tryptophan, leucine and histidine (−TLH), respectively (upper and middle panels). Confirmation of these results was obtained by X-gal filter assay (lower panel). The experiments have been repeated twice with similar outcomes. (b) Yeast two-hybrid analysis of the interaction of NUB1L with individual subunits of the human 19S RP. The yeast two-hybrid analysis was performed as in (a) except that plasmid pGADT7–NUB1L was used instead of pGADT7–FAT10. Figure 1: hRpn10 interacts with FAT10 and NUB1L in a yeast two-hybrid assay. ( a ) Yeast two-hybrid analysis of the interaction of FAT10 with individual subunits of the human 19S RP. AH109 cells were co-transformed with pGADT7–FAT10 and a pGBD vector encoding one of the human 19S RP subunits fused to GAL4-BD. The colonies represent co-transformants with pGADT7–FAT10 and the indicated pGBD construct: (1) S1/Rpn2, (2) S2/Rpn1, (3) S3/Rpn3, (4) S4/Rpt2, (5) S5a/Rpn10, (6) S5b, (7) S6a/Rpt5, (8) S6b/Rpt3, (9) S7/Rpt1, (10) S8/Rpt6, (11) S9/Rpn6, (12) S10a/Rpn7, (13) S10b/Rpt4, (14) S11/Rpn9, (15) S12/Rpn8, (16) S13/Rpn11, (17) S14/Rpn12, (18) S15, (19) p55/Rpn5. (20) As positive control, we co-transformed the NMY51 cells with pGADT7–NUB1L and pLexA–FAT10. A second positive control (21) was the known interaction of NUB1L and hRpn10. Transformants were grown on selection plates containing 3-AT but lacking tryptophan and leucine (−TL) or tryptophan, leucine and histidine (−TLH), respectively (upper and middle panels). Confirmation of these results was obtained by X-gal filter assay (lower panel). The experiments have been repeated twice with similar outcomes. ( b ) Yeast two-hybrid analysis of the interaction of NUB1L with individual subunits of the human 19S RP. The yeast two-hybrid analysis was performed as in ( a ) except that plasmid pGADT7–NUB1L was used instead of pGADT7–FAT10. Full size image FAT10 binds to hRpn10 and NUB1L to hRpn10 and hRpn1 To test whether the interactions of FAT10 and NUB1L with hRpn10 can be attributed to a direct binding of the proteins, glutathione S -transferase (GST)-pull-down experiments were performed. His-hRpn10 showed specific binding to GST–FAT10 and GST–NUB1L, but not to the GST control ( Fig. 2a ) confirming a direct interaction of FAT10 and NUB1L with hRpn10. Moreover, we also found specific binding of the yeast Rpn10 protein (scRpn10) to GST–FAT10 and GST–NUB1L ( Fig. 2b ). 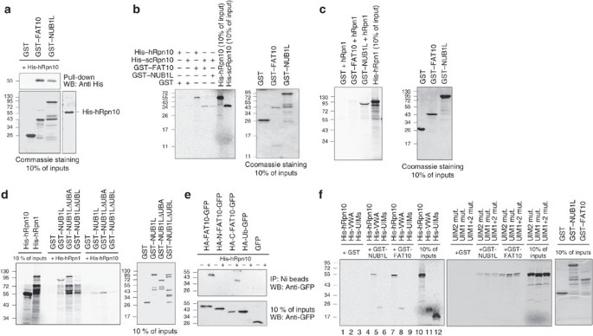Figure 2: Direct interaction of FAT10 and NUB1L with the VWA domain of hRpn10 and binding of hRpn1 by NUB1L. (a) Direct interaction of FAT10 and NUB1L with hRpn10. Recombinant GST, GST–FAT10 or GST–NUB1L was incubated with recombinant His-hRpn10 and GSH beads. The interaction was analysed by western blotting with anti-His antibody. 10% of the recombinant proteins are shown. (b) Interaction of scRpn10 with FAT10 and NUB1L. Recombinant GST, GST–FAT10 or GST–NUB1L was incubated within vitrotranscribed and translated His-hRpn10 or His-scRpn10 along with GSH beads. The interaction of hRpn10 with GST–FAT10 served as positive control. (c) Binding of NUB1L to hRpn1.In vitrotranslated35S-labelled His-hRpn1 was incubated with recombinant GST, GST–FAT10 or GST–NUB1L on GSH beads and the interaction was monitored by autoradiography; 10% of input of the indicated GST-tagged proteins is shown on the right. (d) Binding of NUB1L to hRpn1 requires the UBL domain of NUB1L. GST-pull-down experiments were performed with GST–NUB1LΔUBL or GST–NUB1LΔUBA. (e) The C-terminal UBL domain of FAT10 docks to hRpn10. Co-immunoprecipitation of recombinant His-hRpn10 on Ni-beads with the lysates from HEK 293T cells transfected with the plasmids shown. Positive interaction was determined by immunoblotting with anti-GFP antibody; 10% of the input of proteins was subjected to anti-GFP western blots on the bottom. (f) FAT10 and NUB1L bind to the VWA domain of hRpn10. GST-pull-down experiments with GST–FAT10 or GST–NUB1L or GST alone and within vitrotranslated radiolabelled full-length hRpn10, the VWA domain, or the two UIMs of hRpn10 with wild-type or mutated sequence. Proteins were visualized by autoradiography. 10% of the input of GST-tagged proteins is shown on Coomassie-stained gels to the right. Experiments were repeated three times with similar results. Figure 2: Direct interaction of FAT10 and NUB1L with the VWA domain of hRpn10 and binding of hRpn1 by NUB1L. ( a ) Direct interaction of FAT10 and NUB1L with hRpn10. Recombinant GST, GST–FAT10 or GST–NUB1L was incubated with recombinant His-hRpn10 and GSH beads. The interaction was analysed by western blotting with anti-His antibody. 10% of the recombinant proteins are shown. ( b ) Interaction of scRpn10 with FAT10 and NUB1L. Recombinant GST, GST–FAT10 or GST–NUB1L was incubated with in vitro transcribed and translated His-hRpn10 or His-scRpn10 along with GSH beads. The interaction of hRpn10 with GST–FAT10 served as positive control. ( c ) Binding of NUB1L to hRpn1. In vitro translated 35 S-labelled His-hRpn1 was incubated with recombinant GST, GST–FAT10 or GST–NUB1L on GSH beads and the interaction was monitored by autoradiography; 10% of input of the indicated GST-tagged proteins is shown on the right. ( d ) Binding of NUB1L to hRpn1 requires the UBL domain of NUB1L. GST-pull-down experiments were performed with GST–NUB1LΔUBL or GST–NUB1LΔUBA. ( e ) The C-terminal UBL domain of FAT10 docks to hRpn10. Co-immunoprecipitation of recombinant His-hRpn10 on Ni-beads with the lysates from HEK 293T cells transfected with the plasmids shown. Positive interaction was determined by immunoblotting with anti-GFP antibody; 10% of the input of proteins was subjected to anti-GFP western blots on the bottom. ( f ) FAT10 and NUB1L bind to the VWA domain of hRpn10. GST-pull-down experiments with GST–FAT10 or GST–NUB1L or GST alone and with in vitro translated radiolabelled full-length hRpn10, the VWA domain, or the two UIMs of hRpn10 with wild-type or mutated sequence. Proteins were visualized by autoradiography. 10% of the input of GST-tagged proteins is shown on Coomassie-stained gels to the right. Experiments were repeated three times with similar results. Full size image Recently, it was shown that a conserved amino-terminal region of Rpn13, the Pru domain, binds to ubiquitin and also binds to UBL domains of UBL-UBA proteins like hHR23a and hPLIC2 (ref. 4 ). Although FAT10 failed to bind to the Pru domain of Rpn13 in an earlier study [4] , we re-investigated this possibility with full-length hRpn13 in GST-pull-down assay, and we likewise observed that hRpn13-myc was pulled down neither by GST–FAT10 nor GST–NUB1L. Taking into consideration that the UBL domain of Rad23 and Dsk2 interact with the leucine-rich-repeat-like domain of the Rpn1 subunit of the 19S RP [35] , we hypothesized that FAT10 or NUB1L might also interact with hRpn1. Binding assays with recombinant GST–FAT10, GST–NUB1L or GST alone and radiolabelled in vitro translated His-hRpn1 were carried out. Remarkably, His-hRpn1 bound robustly to GST–NUB1L but did not bind to GST–FAT10 or GST alone ( Fig. 2c ). To test whether NUB1L binding to hRpn1 depended on the UBL domain or the two UBA domains of NUB1L, GST-pull-down experiments with NUB1L-deletion variants were carried out. The deletion of the UBL domain (GST–NUB1LΔUBL) resulted in a strong reduction of His-hRpn1 binding ( Fig. 2d ) indicating a pivotal role of the UBL domain of NUB1L in the binding of His-hRpn1. Moreover, we also investigated whether the UBL domain of NUB1L is essential for the interaction with hRpn10 and, as observed in GST-pull-down assays, the interaction was very weak, if the UBL domain was missing as compared with the interaction when the UBA domains were missing ( Fig. 2d ). Together, our data show that NUB1L binds to hRpn1 and hRpn10 predominantly via its UBL domain. The C-terminal UBL domain of FAT10 interacts with hRpn10 FAT10 consists of two ubiquitin-like domains ( Supplementary Fig. S1 ) [20] . To determine which FAT10 domain interacts with hRpn10, recombinant His-Rpn10 was incubated with lysates from HEK293T cells transiently transfected with the plasmid carrying HA–FAT10-GFP, HA-N-FAT10-GFP, HA-C-FAT10-GFP, HA-Ub-GFP, and GFP alone. Interestingly, only the C-terminal UBL domain of FAT10 bound to hRpn10 but not the N-terminal UBL of FAT10 ( Fig. 2e ); full-length HA–FAT10-GFP served as a positive control and HA-Ub-GFP as well as GFP alone did not show any binding to hRpn10 that served as negative controls. Thus, the N-terminal UBL domain of FAT10 binds to NUB1L [34] , whereas the C-terminal UBL domain binds to hRpn10. FAT10 and NUB1L interact with the VWA domain of hRpn10 As mentioned above, human Rpn10 contains three domains, the VWA domain and two ubiquitin interacting motifs (UIM1 and UIM2). The UIMs are binding sites for polyubiquitin chains [9] , [11] . To identify the domain within the hRpn10 protein mediating FAT10 and NUB1L binding, GST-pull down assays were performed. In vitro translated full-length His-hRpn10 as well as the His-tagged VWA domain alone (His-VWA) bound to GST–FAT10 and GST–NUB1L, whereas no binding was detectable for the two UIMs of hRpn10 ( Fig. 2f ). Polyubiquitin chains bind preferably to UIM2 and to a lesser extent to UIM1 (ref. 12 ). The amino-acid sequence motifs crucial for the binding of polyubiquitin to UIM1 and UIM2 are designated LALAL and IAYAM, respectively [12] . To corroborate the above finding, we performed the same experiment with full-length hRpn10 bearing a mutated LALAL motif in UIM1 (mutated to AAAAA) and a mutated IAYAM motif in UIM2 (mutated to AAAAA; hereafter referred to as mutated UIMs) and observed that FAT10 and NUB1L can still interact with these mutated proteins ( Fig. 2f ). On comparing the amino-acid sequences of FAT10 and ubiquitin, we realized that the key residues within ubiquitin required for binding to the hRpn10 UIM domains, Leu8, Ile44 and Val70 neither align with FAT10's N-terminal nor its C-terminal UBL domain ( Supplementary Fig. S1 ). This observation is in accordance with separate binding sites for FAT10 and ubiquitin within hRpn10. Collectively, our results show that FAT10 and NUB1L bind to the VWA domain of hRpn10 in contrast to polyubiquitin chains that bind to the UIM domains of hRpn10. Rescue of Rpn10Δ yeast with human Rpn10 or the VWA domain The role of hRpn10, in particular that of its VWA domain, in the degradation of FAT10 was investigated in Saccharomyces cerevisiae as Rpn10-deficient yeast is viable. We tested whether hRpn10 can functionally substitute for scRpn10 in S. cerevisiae . Yeast cells lacking Rpn10 ( rpn10 Δ) show a pronounced sensitivity towards canavanine [3] . Canavanine is an arginine analogue causing misfolding of proteins that are targeted for proteasomal degradation. Consistent with an earlier study [3] , N-terminally FLAG-tagged scRpn10 expressed from a high-copy plasmid lead to a suppression of the canavanine sensitivity of rpn10 Δ (NRY5) cells restoring WT-like growth on plates containing 3 μg ml −1 canavanine, whereas the growth of rpn10 Δ cells transformed with an empty plasmid was strongly retarded ( Fig. 3 ). In the same experiment, rpn10 Δ cells transformed with the FLAG-hRpn10 expression construct showed growth on a canavanine containing plate comparable to that of rpn10 Δ cells reconstituted with scRpn10 ( Fig. 3 ), indicating that hRpn10 can functionally substitute for scRpn10 in S. cerevisiae . Earlier studies demonstrated that the rpn10-uim mutant or the VWA domain of Rpn10 show wild-type level of sensitivity to canavanine [18] , [36] . Whether the VWA domain of hRpn10 alone or hRpn10 with mutated UIMs would be able to suppress the canavanine sensitivity of rpn10 Δ cells was tested. Interestingly, expression of both, the FLAG-tagged VWA domain as well as the hRpn10 with mutated UIMs, led to a partial suppression of the canavanine sensitivity ( Fig. 3 ) indicating that the VWA domain alone is able to functionally reconstitute the Rpn10-deficient yeast proteasome. 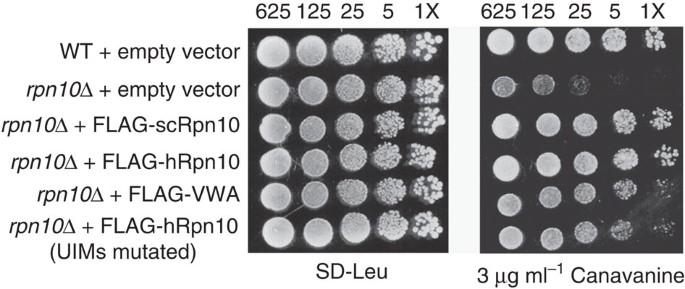Figure 3: Reconstitution of canavanine-resistant growth of scRpn10Δ yeast with hRpn10 or its VWA domain. Canavanine sensitivity plate growth assay with WT andrpn10ΔS. cerevisiaetransformants. WT orrpn10Δ cells transformed with high-copy expression plasmids for FLAG-scRpn10, FLAG-hRpn10, FLAG-VWA or FLAG-hRpn10-UIMs mutated or with the empty plasmid were spotted on plates with synthetic medium lacking leucine (SD-Leu) or on plates lacking leucine and arginine that contain 3 μg ml−1canavanine. The growth assay has been repeated three times with similar results. Figure 3: Reconstitution of canavanine-resistant growth of scRpn10Δ yeast with hRpn10 or its VWA domain. Canavanine sensitivity plate growth assay with WT and rpn10 Δ S. cerevisiae transformants. WT or rpn10 Δ cells transformed with high-copy expression plasmids for FLAG-scRpn10, FLAG-hRpn10, FLAG-VWA or FLAG-hRpn10-UIMs mutated or with the empty plasmid were spotted on plates with synthetic medium lacking leucine (SD-Leu) or on plates lacking leucine and arginine that contain 3 μg ml −1 canavanine. The growth assay has been repeated three times with similar results. Full size image FAT10 binds to the proteasome in wild-type but not rpn10Δ yeast A potential binding of FAT10 with proteasome-associated scRpn10 in yeast was further analysed by glycerol gradient centrifugation. Lysates of either WT or rpn10 Δ cells expressing N-terminally HA-tagged FAT10 were separated by glycerol gradient centrifugation, and collected fractions were analysed by immunoblotting ( Fig. 4a,b ). Free cytosolic Rpn10 was observed in low molecular weight fractions 1–4. Western blots probed with anti-pre6, anti-scRpn10, anti-Rpt1 antibodies showed the presence of 20S and 19S RP in fractions 10–16 and 10–15 in the wild-type and rpn10Δ strains, respectively. We could detect a very low level of RP–CP–RP complex in the fractions from the wild-type yeast (19–20) but not in fractions from rpn10Δ yeast, which is in accordance with the previous studies, which showed the dissociation of lid and the base in the rpn10Δ yeast [6] , [19] . The presence of pre6 and Rpt1 in the same fractions showed their existence in the form of a complex (probably RP–CP complex) in the rpn10Δ yeast strain as well. Aminopeptidase I ( ∼ 600 kDa decamer, AP1) served as a size marker for fractions containing 20S proteasome. In the extract derived from WT cells, HA–FAT10 migrated in the lower and the higher molecular weight fractions (fractions 1–12 and 15–20; Fig. 4a ), whereas it was only found in the lower molecular weight fractions in extracts from cells lacking Rpn10 (fractions 1–8; Fig. 4b ), suggesting the association of FAT10 with proteasome-associated Rpn10. The presence of 20S proteasome in these high molecular weight fractions (fractions 10–15) was further corroborated by the presence of hydrolytic activity towards the fluorogenic substrate Suc-LLVY-AMC ( Fig. 4c ). The peptidase activity increased in the presence of 0.02% SDS indicating the presence of 20S proteasome, whereas the activity was almost abolished in the presence of the proteasome inhibitor MG132 ( Fig. 4c ). 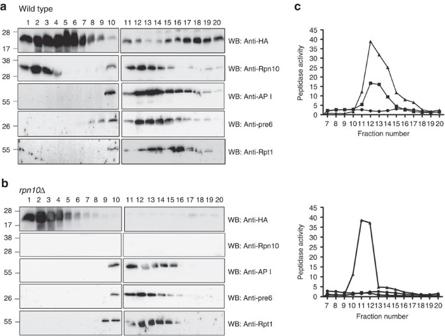Figure 4: Glycerol gradient fraction analysis showing the interaction of FAT10 with the yeast proteasome. (a) Whole-cell lysate from the wild-type yeast transformed with a low-copy plasmid expressing HA–FAT10 was loaded onto a 10–40% glycerol gradient and subjected to ultra-centrifugation (see Methods). The fractions were analysed by western blotting with anti-HA, anti-scRpn10, anti-aminopeptidase I (AP I), anti-pre6 and anti-Rpt1 antibodies. HA–FAT10 migrated to higher fractions of about 600 kDa (fraction 11–12 and 15–20). AP I, which is a decamer of 600 kDa, served as size marker. (b) Glycerol gradient fraction analysis of a whole-cell lysate fromrpn10Δ cells transformed with a low-copy plasmid expressing HA–FAT10. Analysis was performed as in (a). (c) Peptidase activity analysis. The upper graph shows peptidase activity in cell lysates of wild type, the lower graph in cell lysates ofrpn10Δ cells. The fractions of glycerol gradients were analysed for proteolytic activity with the fluorogenic substrate Suc-LLVY-AMC (filled squares). Treatment with MG132 reduced the peptidase activity to basal level (filled circles), which confirmed that this activity relied on the proteasome. After addition of 0.02% SDS, the peptidase activity of 20S proteasome-containing fractions was increased (filled triangles). The unspecific background activity by the substrate was subtracted. Figure 4: Glycerol gradient fraction analysis showing the interaction of FAT10 with the yeast proteasome. ( a ) Whole-cell lysate from the wild-type yeast transformed with a low-copy plasmid expressing HA–FAT10 was loaded onto a 10–40% glycerol gradient and subjected to ultra-centrifugation (see Methods). The fractions were analysed by western blotting with anti-HA, anti-scRpn10, anti-aminopeptidase I (AP I), anti-pre6 and anti-Rpt1 antibodies. HA–FAT10 migrated to higher fractions of about 600 kDa (fraction 11–12 and 15–20). AP I, which is a decamer of 600 kDa, served as size marker. ( b ) Glycerol gradient fraction analysis of a whole-cell lysate from rpn10 Δ cells transformed with a low-copy plasmid expressing HA–FAT10. Analysis was performed as in ( a ). ( c ) Peptidase activity analysis. The upper graph shows peptidase activity in cell lysates of wild type, the lower graph in cell lysates of rpn10 Δ cells. The fractions of glycerol gradients were analysed for proteolytic activity with the fluorogenic substrate Suc-LLVY-AMC (filled squares). Treatment with MG132 reduced the peptidase activity to basal level (filled circles), which confirmed that this activity relied on the proteasome. After addition of 0.02% SDS, the peptidase activity of 20S proteasome-containing fractions was increased (filled triangles). The unspecific background activity by the substrate was subtracted. Full size image The VWA domain of hRpn10 is required for degradation of FAT10 As FAT10 was found to interact with the VWA domain of hRpn10 ( Fig. 2f ), we investigated whether this interaction would have functional relevance for the degradation of FAT10 in vivo . The degradation rate of ectopically expressed HA–FAT10, in WT and rpn10Δ yeast cells, was determined by cycloheximide chase analysis. HA–FAT10 was readily degraded in WT cells with a half-life of ∼ 2 h, whereas it was stable over the 6-h chase period in rpn10 Δ cells ( Fig. 5a ). HA–FAT10 degradation was almost completely restored in rpn10 Δ cells on ectopic expression of either scRpn10 or hRpn10 ( Fig. 5b ). Remarkably, expression of only the VWA domain was sufficient to restore degradation of HA–FAT10 in cells lacking Rpn10 ( Fig. 5c ). Likewise, hRpn10 with mutated UIMs also restored HA–FAT10 degradation to WT-like levels. 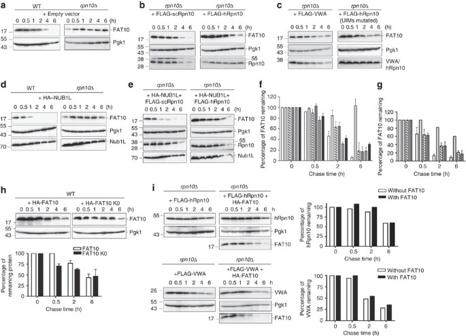Figure 5: Reconstitution of FAT10 degradation in Rpn10-deficient yeast by the VWA domain of hRpn10. Cycloheximide chase analysis of FAT10 stability in WT andrpn10Δ cells reconstituted with hRpn10 or variants and/or NUB1L. HA-tagged FAT10 and NUB1L were visualized by anti-HA western blotting whereas FLAG-tagged proteins, scRpn10, hRpn10, VWA and hRpn10-mutated UIMs were detected via FLAG-specific antibodies. Pgk1 served as a loading control. (a) HA–FAT10 degradation in WT andrpn10Δcells. The experiment was repeated three times with similar outcome (quantitation is shown in (f)). (b) FAT10 degradation inrpn10Δyeast reconstituted with FLAG-scRpn10 (left) or FLAG-hRpn10 (right). (c) FAT10 degradation inrpn10Δyeast reconstituted with FLAG-VWA (left) or FLAG-hRpn10-UIMs mutated (right). (d) Accelerated FAT10 degradation in the presence of NUB1L in wild-type but notrpn10Δyeast. (e) Accelerated FAT10 degradation in the presence of NUB1L inrpn10Δyeast reconstituted with FLAG-scRpn10 (left) or FLAG-hRpn10 (right). (f, g) Quantitation of HA–FAT10 cycloheximide chase experiments in the absence of NUB1L (f) and in the presence of NUB1L (g); WT+empty vector (white),rpn10Δ+empty vector (light grey),rpn10Δ+scRpn10 (hatched),rpn10Δ+hRpn10 (dark grey),rpn10Δ+VWA (dotted),rpn10Δ+hRpn10 with UIMs mutated (black). Values represent the mean±s.e.m. from three experiments (f) and the means±the range from two (g) experiments (h) Degradation of FAT10 in yeast is independent of ubiquitin. Cyloheximide chase was performed after transformation of wild-type yeast with either FAT10 or lysine-deficient FAT10, where all lysines are replaced by arginines (FAT10 K0). The graph represents the mean value±range from two sets of experiments. (i) No effect of FAT10 on the degradation of full-length hRpn10 (top) or the isolated VWA domain (bottom) of hRpn10. Cycloheximide chase experiments were performed for 6 h inrpn10Δyeast reconstituted with FLAG-hRpn10 or FLAG-VWA with and without HA–FAT10 as indicated. Pgk1 western blots served as loading controls. The anti-FLAG western blots and their quantitative evaluations show that the degradation of hRpn10 and VWA is independent of FAT10 expression. Figure 5: Reconstitution of FAT10 degradation in Rpn10-deficient yeast by the VWA domain of hRpn10. Cycloheximide chase analysis of FAT10 stability in WT and rpn10 Δ cells reconstituted with hRpn10 or variants and/or NUB1L. HA-tagged FAT10 and NUB1L were visualized by anti-HA western blotting whereas FLAG-tagged proteins, scRpn10, hRpn10, VWA and hRpn10-mutated UIMs were detected via FLAG-specific antibodies. Pgk1 served as a loading control. ( a ) HA–FAT10 degradation in WT and rpn10Δ cells. The experiment was repeated three times with similar outcome (quantitation is shown in ( f )). ( b ) FAT10 degradation in rpn10Δ yeast reconstituted with FLAG-scRpn10 (left) or FLAG-hRpn10 (right). ( c ) FAT10 degradation in rpn10Δ yeast reconstituted with FLAG-VWA (left) or FLAG-hRpn10-UIMs mutated (right). ( d ) Accelerated FAT10 degradation in the presence of NUB1L in wild-type but not rpn10Δ yeast. ( e ) Accelerated FAT10 degradation in the presence of NUB1L in rpn10Δ yeast reconstituted with FLAG-scRpn10 (left) or FLAG-hRpn10 (right). ( f, g ) Quantitation of HA–FAT10 cycloheximide chase experiments in the absence of NUB1L ( f ) and in the presence of NUB1L ( g ); WT+empty vector (white), rpn10Δ +empty vector (light grey), rpn10Δ +scRpn10 (hatched), rpn10Δ +hRpn10 (dark grey), rpn10Δ +VWA (dotted), rpn10Δ +hRpn10 with UIMs mutated (black). Values represent the mean±s.e.m. from three experiments ( f ) and the means±the range from two ( g ) experiments ( h ) Degradation of FAT10 in yeast is independent of ubiquitin. Cyloheximide chase was performed after transformation of wild-type yeast with either FAT10 or lysine-deficient FAT10, where all lysines are replaced by arginines (FAT10 K0). The graph represents the mean value±range from two sets of experiments. ( i ) No effect of FAT10 on the degradation of full-length hRpn10 (top) or the isolated VWA domain (bottom) of hRpn10. Cycloheximide chase experiments were performed for 6 h in rpn10Δ yeast reconstituted with FLAG-hRpn10 or FLAG-VWA with and without HA–FAT10 as indicated. Pgk1 western blots served as loading controls. The anti-FLAG western blots and their quantitative evaluations show that the degradation of hRpn10 and VWA is independent of FAT10 expression. Full size image NUB1L relies on hRpn10 for promoting the degradation of FAT10 Because the degradation of FAT10 is accelerated by NUB1L [32] , and because both FAT10 and NUB1L interact with hRpn10, we investigated whether the stimulating effect of NUB1L on the degradation of FAT10 would depend on hRpn10 in vivo . Cycloheximide chase experiments were performed as described above, except that HA–NUB1L was also expressed in yeast cells. The HA–FAT10 protein remained stable in rpn10Δ yeast cells even in the presence of HA–NUB1L, but its degradation was accelerated in wild-type cells ( Fig. 5d ). Following reconstitution of HA–NUB1L expressing rpn10Δ cells with either FLAG-scRpn10 or FLAG-hRpn10, degradation rates similar to that of the WT strain expressing HA–NUB1L were observed ( Fig. 5e–g ; Supplementary Fig. S2 ). The quantitative analysis revealed that the half-life of HA–FAT10 was reduced to less than 1 h ( Fig. 5g ). Collectively, these results show that the accelerating effect of NUB1L on FAT10 degradation is dependent on hRpn10. To confirm the earlier finding that the degradation of FAT10 is independent of ubiquitin [21] , [22] , we analysed the degradation of lysine-deficient FAT10 in yeast and found it to be degraded as rapidly as WT FAT10 ( Fig. 5h ). We noted that FLAG-hRpn10 or FLAG-VWA was also degraded over time ( Fig. 5b,c ) but this degradation occurred independently of HA–FAT10 ( Fig. 5i ). Degradation of FAT10 via hRpn10-VWA is proteasome-dependent To determine whether FAT10 is degraded by the proteasome, we investigated whether FAT10 could be stabilized by MG132 (ref. 37 ). The pdr5 gene was disrupted in WT and rpn10 Δ cells, as WT yeast cells readily export MG132 via the multi-drug transporter Pdr5 rendering them resistant to MG132. Cycloheximide chase experiments in the presence of MG132 were performed in pdr5Δ (NRY51) and pdr5Δrpn10Δ (NRY53) cells transformed with an expression plasmid for HA–FAT10 alone or in combination with an expression plasmid for FLAG-hRpn10 or FLAG-VWA. Strikingly, addition of MG132 led to a strong stabilization of FAT10 in all the transformants tested, even in the pdr5 Δ rpn10 Δ strain reconstituted with only the VWA domain ( Fig. 6a–c ). Additionally, the degradation of FAT10 was analysed in the proteasome mutant yeast strain pre1-1 (ref. 38 ). Cycloheximide chase experiments were performed after transforming HA–FAT10 into pre1-1 and its parental strain. We observed the stabilization of FAT10 in pre1-1 strain as compared with the WT strain under non-permissive conditions ( Fig. 6d ). Moreover, mutating the Asp11 residue in the VWA domain of human or yeast Rpn10 to Ala, which affects ubiquitin-mediated proteolysis by the 26S proteasome, also interferes with the degradation of FAT10 ( Supplementary Fig. S3 ). Taken together, these data strongly suggests that the degradation of FAT10 is proteasome-dependent. 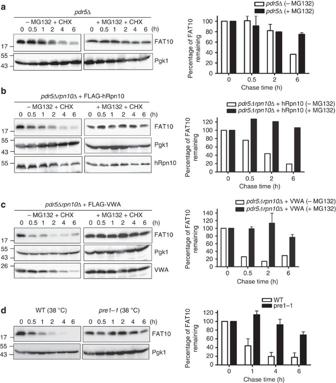Figure 6: The degradation of FAT10in vivois dependent on proteasome activity. (a) HA–FAT10 cycloheximide chase analysis inpdr5Δyeast cells in the presence or absence of the proteasome inhibitor MG132 with quantitative analysis of the densities of HA–FAT10 bands in the western blot. (b) Cycloheximide chase analysis withpdr5Δrpn10Δ cells ectopically expressing FLAG-hRpn10; western blots on the bottom monitor FLAG-hRpn10 levels. (c) Cycloheximide chase analysis withpdr5Δrpn10Δ cells ectopically expressing FLAG-VWA; western blots on the bottom monitor FLAG-VWA expression. (d) Cycloheximide chase analysis of the degradation of HA–FAT10 in wild type (WCG4a) and the proteasome subunit mutantpre1-1yeast strain with quantitative analysis of HA–FAT10 western blots. Pgk1 western blots served as loading controls in all panels. The graphs represent the mean value±range from two independent sets of experiments. Figure 6: The degradation of FAT10 in vivo is dependent on proteasome activity. ( a ) HA–FAT10 cycloheximide chase analysis in pdr5Δ yeast cells in the presence or absence of the proteasome inhibitor MG132 with quantitative analysis of the densities of HA–FAT10 bands in the western blot. ( b ) Cycloheximide chase analysis with pdr5 Δ rpn10 Δ cells ectopically expressing FLAG-hRpn10; western blots on the bottom monitor FLAG-hRpn10 levels. ( c ) Cycloheximide chase analysis with pdr5 Δ rpn10 Δ cells ectopically expressing FLAG-VWA; western blots on the bottom monitor FLAG-VWA expression. ( d ) Cycloheximide chase analysis of the degradation of HA–FAT10 in wild type (WCG4a) and the proteasome subunit mutant pre1-1 yeast strain with quantitative analysis of HA–FAT10 western blots. Pgk1 western blots served as loading controls in all panels. The graphs represent the mean value±range from two independent sets of experiments. Full size image FAT10 competes with NUB1L for binding to hRpn10-VWA As mentioned above, the N-terminal domain of FAT10 docks to NUB1L [34] , whereas the C-terminal domain of FAT10 docks to hRpn10 ( Fig. 2e ). To investigate whether a trimeric complex is formed, GST–NUB1LΔUBL bound to glutathione-sepharose (reduced) beads was incubated with His-hRpn10 and FAT10 either in equimolar amount or with increasing concentrations. An increase in the binding of His-hRpn10 on the beads with the increasing concentrations of FAT10 was clearly observed ( Fig. 7a ), which confirmed that FAT10 can bind to NUB1L and hRpn10 simultaneously using distinct domains. 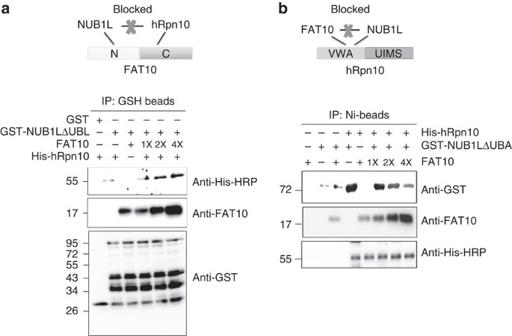Figure 7: Trimeric complex formation and competition between FAT10 and NUB1L for hRpn10. (a) Trimeric complex formation. 60 pmol of recombinant GST or GST–NUB1LΔUBL was precipitated on GSH-sepharose beads and incubated with 30 pmol of His-hRpn10 (lane 2) either alone or together with 60 pmol or increasing molar excess of FAT10 (lane 4, 5 and 6). After incubation for 2 h at 4 °C, the beads were washed and the interaction was analysed by western blotting with anti-His-HRP, anti-FAT10 and anti-GST antibodies. (b) 30 pmol of recombinant His-Rpn10 was precipitated on Ni-beads and incubated with 60 pmol of GST–NUB1LΔUBA in the absence or presence of FAT10 (lane 4–8). FAT10 was added in increasing molar excesses as indicated in lane 7 and 8. The binding of NUB1LΔUBA during the course of competition was analysed by western blotting. The experiments have been repeated at least twice with similar results. Figure 7: Trimeric complex formation and competition between FAT10 and NUB1L for hRpn10. ( a ) Trimeric complex formation. 60 pmol of recombinant GST or GST–NUB1LΔUBL was precipitated on GSH-sepharose beads and incubated with 30 pmol of His-hRpn10 (lane 2) either alone or together with 60 pmol or increasing molar excess of FAT10 (lane 4, 5 and 6). After incubation for 2 h at 4 °C, the beads were washed and the interaction was analysed by western blotting with anti-His-HRP, anti-FAT10 and anti-GST antibodies. ( b ) 30 pmol of recombinant His-Rpn10 was precipitated on Ni-beads and incubated with 60 pmol of GST–NUB1LΔUBA in the absence or presence of FAT10 (lane 4–8). FAT10 was added in increasing molar excesses as indicated in lane 7 and 8. The binding of NUB1LΔUBA during the course of competition was analysed by western blotting. The experiments have been repeated at least twice with similar results. Full size image As both FAT10 and NUB1L can bind to the VWA domain of hRpn10 ( Fig. 2f ), we determined whether they can compete with each other for hRpn10 binding. To this aim, we utilized a deletion mutant of NUB1L lacking UBA domains, which cannot bind to FAT10 but still binds to hRpn10. Recombinant His-hRpn10 was bound to Ni-beads and recombinant GST–NUB1LΔUBA was incubated with these beads along with FAT10 at increasing concentrations. Interestingly, increasing levels of FAT10 molecules displaced NUB1L from hRpn10 ( Fig. 7b ), which suggests that NUB1L and FAT10 bound to the same motif on the VWA domain implying that, with an excess of FAT10, NUB1L is unable to bind to hRpn10 but can still bind to Rpn1. hRpn10 knockdown in human cells causes FAT10 accumulation Contrary to yeast, mammalian cells deficient in hRpn10 are not viable over extended periods of time [39] , [40] . Therefore, the function of hRpn10 in the degradation of FAT10 and its conjugates in mammalian cells was addressed by transiently knocking down hRpn10 with short interfering RNA (siRNA) in HEK293 cells that lead to extensive depletion of hRpn10 ( Fig. 8a ) but did not affect their viability during the course of the experiment. The steady-state level of monomeric FAT10, as well as FAT10 conjugates, was significantly increased in cells treated with hRpn10 siRNA as compared with cells treated with control siRNA ( Fig. 8a,b ). In HEK293 cells stimulated with IFN-γ and TNF-α to induce endogenous FAT10 expression, there was no accumulation of FAT10 or FAT10 conjugates when normalized to β -actin expression ( Fig. 8c ). However, real-time RT–PCR analysis revealed that treatment of cytokine-induced cells with hRpn10 siRNAs consistently reduced endogenous FAT10 messenger RNA levels by ∼ 60% when compared with cells treated with control siRNA ( Fig. 8d ). When we normalized the levels of monomeric or substrate-conjugated endogenous FAT10 protein on the level of FAT10 mRNA, we confirmed an accumulation of FAT10 and its conjugates after knockdown of hRpn10 ( Fig. 8d ). 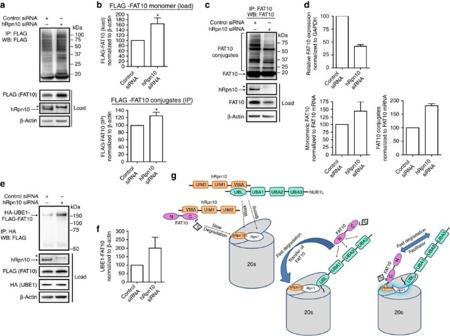Figure 8: Knockdown of hRpn10 in HEK293 cells causes accumulation of FAT10 and FAT10 conjugates. (a) HEK293 cells were transfected with hRpn10 or control siRNA and His-3×FLAG-FAT10 (FLAG-FAT10). Lysates were immunoprecipitated with anti-FLAG-sepharose. A western blot of immunoprecipitated FLAG-FAT10 and indicated proteins in lysates (load) are shown. Asterisks mark unspecific signals. (b) Quantification of monomeric and conjugated FAT10 in (a) normalized to β-actin. Significance was calculated with paired two-tailP-value test. Values represent the mean±s.e.m. of 9 (monomeric FAT10) and 7 (FAT10 conjugates) experiments. (c) Accumulation of endogenous FAT10 upon downregulation of hRpn10. HEK293 cells were treated with control or hRpn10 siRNA and 24 h later with IFN-γ/TNF-α for extra 24 h. FAT10 immunoprecipitates were analysed by western blot with a polyclonal FAT10-reactive antibody (top) and expression levels of hRpn10, endogenous FAT10, and β-actin in lysates are shown (below). One of three experiments with similar outcome is shown. (d) Induction of endogenousFAT10expression was measured by real-time RT–PCR, RNA levels were normalized toGAPDH. The mean of three independent experiments is shown. Signals for monomeric (load) and conjugated FAT10 (IP) were normalized to FAT10 mRNA levels. (e) Western blot showing accumulation of UBE1–FAT10 conjugate upon downregulation of hRpn10. HEK293 cells were transfected with hRpn10 or control siRNAs and His-3×FLAG-FAT10 (FLAG-FAT10) and HA-UBE1 plasmids. Western blots of HA immunoprecipitates (top) and indicated proteins in total lysates (load) are shown. A representative experiment out of three is shown. (f) Signals of three experiments as in (e) were quantified and normalized to β-actin. Values represent mean±s.e.m. of three experiments. (g) Models of FAT10 and NUB1L-mediated degradation by the 26S proteasome. (Top) Slow degradation of FAT10 conjugates by the 26S proteasome when interacting with the VWA domain of hRpn10 in the absence of NUB1L. (Bottom left) Transfer model showing accelerated degradation of FAT10 when NUB1L interacts with hRpn1 and the N-terminal UBL domain of FAT10, which is subsequently transferred to hRpn10. (Bottom right) Facilitator model: FAT10 docks onto hRpn10 while its degradation is facilitated by binding of NUB1L to hRpn1 leading to conformational changes in both subunits. Figure 8: Knockdown of hRpn10 in HEK293 cells causes accumulation of FAT10 and FAT10 conjugates. ( a ) HEK293 cells were transfected with hRpn10 or control siRNA and His-3×FLAG-FAT10 (FLAG-FAT10). Lysates were immunoprecipitated with anti-FLAG-sepharose. A western blot of immunoprecipitated FLAG-FAT10 and indicated proteins in lysates (load) are shown. Asterisks mark unspecific signals. ( b ) Quantification of monomeric and conjugated FAT10 in ( a ) normalized to β-actin. Significance was calculated with paired two-tail P -value test. Values represent the mean±s.e.m. of 9 (monomeric FAT10) and 7 (FAT10 conjugates) experiments. ( c ) Accumulation of endogenous FAT10 upon downregulation of hRpn10. HEK293 cells were treated with control or hRpn10 siRNA and 24 h later with IFN-γ/TNF-α for extra 24 h. FAT10 immunoprecipitates were analysed by western blot with a polyclonal FAT10-reactive antibody (top) and expression levels of hRpn10, endogenous FAT10, and β-actin in lysates are shown (below). One of three experiments with similar outcome is shown. ( d ) Induction of endogenous FAT10 expression was measured by real-time RT–PCR, RNA levels were normalized to GAPDH . The mean of three independent experiments is shown. Signals for monomeric (load) and conjugated FAT10 (IP) were normalized to FAT10 mRNA levels. ( e ) Western blot showing accumulation of UBE1–FAT10 conjugate upon downregulation of hRpn10. HEK293 cells were transfected with hRpn10 or control siRNAs and His-3×FLAG-FAT10 (FLAG-FAT10) and HA-UBE1 plasmids. Western blots of HA immunoprecipitates (top) and indicated proteins in total lysates (load) are shown. A representative experiment out of three is shown. ( f ) Signals of three experiments as in ( e ) were quantified and normalized to β-actin. Values represent mean±s.e.m. of three experiments. ( g ) Models of FAT10 and NUB1L-mediated degradation by the 26S proteasome. (Top) Slow degradation of FAT10 conjugates by the 26S proteasome when interacting with the VWA domain of hRpn10 in the absence of NUB1L. (Bottom left) Transfer model showing accelerated degradation of FAT10 when NUB1L interacts with hRpn1 and the N-terminal UBL domain of FAT10, which is subsequently transferred to hRpn10. (Bottom right) Facilitator model: FAT10 docks onto hRpn10 while its degradation is facilitated by binding of NUB1L to hRpn1 leading to conformational changes in both subunits. Full size image Recently, we have identified the ubiquitin-activating enzyme UBE1 as a substrate of FAT10ylation, and we tested whether the UBE1–FAT10 conjugate would accumulate in HEK293 cells upon hRpn10 knockdown. Depletion of hRpn10 led to a twofold increase in the amount of UBE1–FAT10 conjugate ( Fig. 8e, f ). These results suggest that hRpn10 functions as a receptor for FAT10 and its conjugates and targets them for proteasomal degradation also in mammalian cells. Degradation of proteins by the proteasome is regulated at several levels. One level is the docking step to the 26S proteasome, which in the ubiquitin system, is mediated by binding of poly-ubiquitin chains to the proteasome subunits Rpn10 or Rpn13 or to soluble ubiquitin receptors, which in turn bind to Rpn1 or Rpn2 (ref. 1 ). Interestingly, these two binding modes seem to mutually affect each other, as the degradation of poly-ubiquitylated Sic1 at the isolated 26S proteasome via Rad23 was shown to be facilitated by binding of the VWA domain of the Rpn10 subunit to the proteasome [19] . Similar evidence regulating the pace of proteasomal degradation has been observed for the FAT10 system where NUB1L accelerated FAT10 degradation about eightfold [32] . This stimulating effect relied on the N-terminal UBL domain of NUB1L required for proteasome binding and was independent of the three UBA domains of NUB1L, which bind to FAT10 (ref. 34 ). FAT10, therefore, resembles ubiquitin in that it can bind directly to the proteasome or can become tethered to the proteasome via the UBL–UBA protein NUB1L. To better understand how NUB1L influences the rate of FAT10 degradation, we set out to identify the subunit(s) of the RP which bind to FAT10. Rpn10 was the only RP subunit found to interact with FAT10 in our yeast two-hybrid analysis. The finding that FAT10 and NUB1L bind to the same subunit raised the question how NUB1L may act as a facilitator of FAT10-mediated degradation. One possibility was that FAT10 and NUB1L bind to different domains of Rpn10. It was therefore surprising that both of them bound to the same domain. Even more surprising was that these two ubiquitin-like proteins did not bind to the UIM domains of Rpn10, like ubiquitin, but instead to the VWA domain, which seems to be a novel UBL-binding domain ( Fig. 2f ). VWA domains contain a β-sheet sandwiched by multiple α-helices and they usually bind to metal ions via a metal ion-dependent adhesion site. It was hypothesized that the VWA domains mediate protein–protein interactions involved in the assembly or function of multi-protein complexes [7] , [36] . We have extensively tried to identify the residues within the VWA domain that are involved in FAT10- and NUB1L-binding by mutagenesis. However, several combined point mutations were unsuccessful in abolishing the binding to NUB1L or FAT10, whereas deletion variants could not be stably expressed. The human Rpn10 subunit was able to reconstitute growth of rpn10Δ S. cerevisiae cells in canavanine sensitivity assays ( Fig. 3 ). Rpn10 is required to keep the base and the lid of the RP firmly associated [6] , [19] and our transcomplementation data with human Rpn10 suggest that the human orthologue can serve this structural function also in the context of the yeast 26S proteasome. The reconstitution of Rpn10-deficient yeast with human Rpn10 encouraged us to test whether FAT10 degradation could be reconstituted in yeast. The reconstitution of FAT10 degradation in yeast seemed justified as Rpn10 has been shown to be essential in mouse cells [40] and is required for normal degradation of ubiquitin-conjugates in Drosophila [39] . We could show that FAT10 is degraded in yeast in a Rpn10-dependent manner ( Fig. 5 ). The fact that FAT10 degradation was supported by both yeast and human Rpn10 is consistent with the finding that not the UIMs (which differ in number between human and yeast), but the VWA domain of Rpn10 is required for FAT10 degradation. This system further allowed us to show that the VWA domain sufficed to robustly reconstitute FAT10 degradation ( Fig. 5c ), which is in accordance with our binding studies ( Fig. 2f ). Interestingly, the VWA domain could largely restore wild-type-like growth of Rpn10-deficient yeast on canavanine-containing plates ( Fig. 3 ). Consistently, mice bearing only a VWA domain survive longer than mice that completely lack mRpn10 (ref. 40 ). The knockdown of hRpn10 in human HEK293 cells led to an accumulation of FLAG–FAT10 and endogenous FAT10 and bulk FAT10 conjugates (when normalized to the level of FAT10 mRNA), and the UBE1–FAT10 conjugate by 30–50% ( Fig. 8 ), suggesting that hRpn10 serves as a FAT10 receptor also in humans, although the effect was not as strong as found after rpn10 deletion in yeast. This difference is most likely due to residual hRpn10 protein in the siRNA-treated human cells. Previously the only subunit known to interact with NUB1L was hRpn10 and it was shown that the C terminus of NUB1L binds to hRpn10 (ref. 33 ). Another study reported that the association of NUB1L with the 26S proteasome occurs via the N-terminal UBL domain [34] . We show here that the UBL domain of NUB1L binds to hRpn1 as well as hRpn10 of the 26S proteasome in accordance with the latter report ( Fig. 2d ). Interestingly, we could also show that the C-terminal UBL domain of FAT10 binds to hRpn10 ( Fig. 2e ), which leaves the N-terminal UBL domain of FAT10 free for docking to the UBA domains of NUB1L [34] resulting in formation of a trimeric NUB1L–FAT10–Rpn10 complex ( Fig 7a ). One may speculate about the biological consequences of FAT10 being degraded slowly in the absence of NUB1L and faster in its presence. It is possible that different FAT10ylated substrates require different rates of proteasome-mediated degradation and that only those are bound by NUB1L, which require rapid degradation. A striking difference between ubiquitin and FAT10 is that ubiquitin is recycled with the help of numerous ubiquitin-deconjugating enzymes whereas such enzymes have not been found to date for FAT10 that seems to be degraded along with its substrates [21] , [22] . The overexpression of FAT10 is toxic to cells [27] and it is possible that NUB1L contributes to keeping FAT10 at a low level. The key findings of this study can be exploited to suggest two models for how NUB1L accelerates the degradation of FAT10. FAT10 might directly bind to the VWA domain of hRpn10 and become degraded at a slow rate in the absence of NUB1L ( Fig. 8g ). If NUB1L binds to the Rpn1 subunit, it may act like a soluble 'FAT10-receptor', and transfer-bound FAT10 and its conjugated substrates to the hRpn10 subunit of the proteasome to be degraded faster ( Fig. 8g , transfer model). Alternatively, NUB1L binding to Rpn1 could induce a conformational change in the hRpn10 subunit ( Fig. 8g , facilitator model), which allows FAT10 and its conjugated substrates to be more rapidly degraded. Yeast strains and plasmids Yeast strains and plasmid cloning are described in Supplementary Tables S1 and S2 , respectively. GST-pull-down-assay GST, GST–FAT10, GST–NUB1L, GST–NUB1LΔUBA, GST–NUB1LΔUBL ( Supplementary Table S2 ) and His-hRpn10 (ref. 12 ) (kindly provided by Patrick Young, Stockholm University) were expressed in Escherichia coli strain B834(DE3)pLysS as described [32] . Glutathione sepharose 4B beads (GE Healthcare) were incubated with GST, GST–FAT10 or GST–NUB1L along with purified His-hRpn10 in incubation buffer (20 mM Tris–HCl, pH 7.4, 0.1% TritonX-100) overnight at 4 °C and washed 5 times with incubation buffer. For other experiments, His-hRpn10, His-UIM1+UIM2 domains and His-VWA domain were in vitro transcribed and translated using TNT T7 coupled reticulocyte lysate system (Promega) and purified GST, GST–FAT10 or GST–NUB1L bound on the GSH beads was added. Proteins were eluted by boiling at 95 °C for 5 min with SDS buffer, resolved by SDS–PAGE and subjected to western blot analysis using anti-His antibody (1 μg ml −1 , Sigma) or autoradiography. Yeast strain construction Gene inactivations were performed by transforming yeast with the LiOAc method with a PCR product that encoded either G418 resistance or hygromycin resistance, and contained 40 bp homologous flanking regions. For the construction of rpn10 Δ::KanMX6 allele, the pFA6a-KanMX6 (ref. 41 ) plasmid was used as template for amplification of the KanMX6 cassette and plasmid pAG32 (ref. 42 ) was used for construction of the pdr5 Δ::hphMX4 allele. Following transformation, cells were plated on YPD medium, incubated for ∼ 12 h and were replica-plated onto YPD supplemented with 300 μg ml −1 G418 or 250 μg ml −1 hygromycin B. Canavanine sensitivity assay Wild-type yeast (MHY500) was transformed with empty vector (YEplac181), and the rpn10Δ yeast strain (NRY5) was transformed with empty plasmid (YEplac181) or YEplac181 containing FLAG-scRpn10, FLAG-hRpn10, FLAG-VWA or FLAG-hRpn10 (UIMs-mutated) and plated on selective plates lacking leucine. After 3 days, single transformants were selected and inoculated in synthetic media lacking leucine. Cells were grown to log phase (OD 600 ∼ 1.0), serially diluted (fivefold steps) and spotted on selective plates lacking either leucine (control) or arginine and leucine (with 3 μg ml −1 canavanine). Plates were incubated at 30 °C for 5 days. Glycerol gradient centrifugation Wild-type and rpn10Δ yeast cells transformed with plasmid p414Met25–FAT10 were grown in selective medium to an OD 600 of 3.0. Cell pellets were resuspended in lysis buffer (10% glycerol, 50 mM Tris–HCl, pH 7.4, 10 mM MgCl 2 , 2 mM ATP, 0.5 mM DTT, 100 mM NaCl and protease inhibitors), and lysed using French press. The supernatant from the lysed cells was loaded onto a 10–40% glycerol gradient prepared in lysis buffer. The tubes were ultracentrifuged at 304,660 g for 16 h at 4 °C. 600 μl fractions were collected, and proteins were precipitated by the methanol–chloroform method. Proteins were resolved on SDS–PAGE and blotted with anti-HA-7 (1 μg ml −1 ), anti-AP I (pAb kindly provided by Michael Thumm, Göttingen University), anti Rpn10 (1 μg ml −1 , Abcam), anti-pre6 (pAb, kind gift from Wolfgang Heinemeyer, TU Munich, Germany), anti-Rpt1 (1 μg ml −1 , Enzo Lifesciences) antibodies. For the peptidase activity assay, 20 μl of each fraction was added to 100 μl of Suc-LLVY-AMC (Bachem) with a final concentration of 100 μM in a black 96-well plate and incubated at 37 °C for 30 min. The peptidase activity was recorded with a Tecan SpectraFluor Plus instrument (excitation λ =360 nm, emission λ =465 nm). Cycloheximide chase Cycloheximide (0.25 mg ml −1 ) was added to logarithmically growing yeast cultures (30 °C), and aliquots were removed at indicated times. The experiment with pre1-1 strain (kindly provided by Wolfgang Heinemeyer) was performed as described earlier [38] . Lysates were prepared using the NaOH lysis method [43] and boiled for 5 min. HA–FAT10 (cloned in p416Met25 vector) and HA–NUB1L (cloned in p414GPD vector) were visualized by western blotting with an anti-HA-7 (1 μg ml −1 , Sigma) antibody, hRpn10 and variants (cloned in YEplac181 vector) were detected using an anti-FLAG-HRP antibody (0.5 μg ml −1 , Sigma). Protein degradation after immunoblotting was quantified using Quantity One software (Bio-Rad) and normalized using an anti-Pgk1 (0.1 μg ml −1 , Invitrogen) loading control. Site-directed mutagenesis Oligonucleotide primers were designed complementary to the opposite strands of the vector with the desired mutation: primers for the D11 mutation in the VWA domain in hRPN10: FP: 5′-GGTGTGTGTGGCCAACAGTGAG TATATGCGGAATGG-3′; RP: 5′-CCATTCCGCATATACTCACTGTTGGC CACACACACC-3′; primers for the D11 mutation in the VWA domain in scRpn10: FP: 5′-GCTACAGTGTTAGTGATTGCTAATTCAGAGTACTCTCG-3′; RP: 5′-TGTAGCCGAGAGTACTCTGAATTAGCAATCACTAACAC-3′. The extension of primers by Phusion polymerase generated a plasmid with desired mutation containing staggered nicks. The cycling reaction included denaturation cycle at 95 °C for 30 s; and 12–18 (depending on the number of mutations) cycles at 95 °C for 30 s, 55 °C for 1 min and 68 °C for 5 min. Following PCR cycles, the product was treated with Dpn I enzyme. The vector was transformed into competent cells and isolated plasmids from bacterial colonies were sequenced. Proteasome inhibition A PDR5Δ yeast strain was used for the experiments. The proteasome inhibitor MG132 (Sigma) was added to a final concentration of 70 μM to the cultures before the start of the cycloheximide chase [44] . Fresh MG132 was added every 90 min during the course of the experiment. FAT10 stability was visualized via immunoblotting with an anti-HA antibody (1 μg ml −1 ). Competition assay Ni-beads (EZview His beads, Sigma), blocked with 1 mg ml −1 of BSA, were loaded with 30 pmol of purified His-Rpn10 and resuspended in PBS. The beads were incubated with 60 pmol of purified GST–NUB1LΔUBA in the presence or absence of the competitor FAT10 (purified). For negative controls (lane 1–3), 20 μg of His-peptide (Abcam) was added. After 2 h of binding at 4 °C, the resin was washed three times with NET-TON buffer [23] , two times with NET-T buffer [23] and once with 20 mM Tris buffer (pH 7.8). Bound proteins were analysed by western blotting. Transfection of HEK 293T Cells and Co-immunoprecipitation Complementary DNAs were transfected into HEK 293T cells; cells were washed, and lysed in 250 μl of 50 mM Tris–HCl (pH 7.8) and 0.1% TritonX-100. After centrifugation, the expression of proteins was determined by fluorescence measurement (485 nm excitation, 535 nm emission) in the supernatant. 100 μl Ni-beads (Sigma) and 5 μg recombinant purified His-hRpn10 were incubated overnight at 4 °C in PBS containing 650 mM NaCl, 0.2% Triton X-100 and 1 mg ml −1 methylated BSA. Equal aliquots of lysate were incubated with the Ni-precipitated His-hRpn10 or Ni-beads only. After overnight incubation, the beads were washed 5 times with PBS containing 650 mM NaCl, 0.2% TritonX-100, and once with 5 mM Tris (pH 7.5). Detection of the load and precipitated proteins was performed by western blotting with an anti-GFP-antibody (clone MMS-118P) and the bound His-hRpn10 was detected with an anti-Rpn10 antibody (1 μg ml −1 , Abcam). For induction of endogenous FAT10 expression, HEK293 cells were transfected with control or hRpn10-specific siRNA and after 24 h stimulated with 200 U ml −1 IFN-γ and 400 U ml −1 TNFα for extra 24 h (both from Peprotech). Cells were lysed and subjected to immunoprecipitation using a FAT10 specific mAb (4F1) [23] for immunoprecipitation and a FAT10-reactive polyclonal antibody [21] for western blot analysis. hRpn10 knockdown siRNA transfection was performed as recently described [23] . Briefly, 1.6×10 6 HEK293 cells were transfected with a pool of 3 different human hRpn10-specific siRNAs (Hs_PSMD4_5, Hs_PSMD4_6, Hs_PSMD4_10, Qiagen) or with a negative control siRNA (AllStars Negative Control siRNA, Qiagen) using X-tremeGENE siRNA Transfection Reagent (Roche). Cells were transfected with a total amount of 240 nM siRNA. After 24 h, cells were transfected with the plasmid pcDNA3.1–3×FLAG-His-FAT10 alone or together with pcDNA3.1-HA-UBE1 using TransIT-LT1 transfection reagent (Mirus). After 24 h of incubation, cells were collected and lysates were used for an anti-FLAG or anti-HA immunoprecipitation using 30 μl of EZview Red ANTI-FLAG M2 or anti-HA (HA-7) agarose (Sigma). Western Blot analysis was performed with a direct peroxidase-labelled anti-FLAG-M2-HRP (0.5 μg ml −1 ), a direct peroxidase-labelled anti-HA-7-HRP (1 μg ml −1 , both from SIGMA), an anti-hRpn10 mouse mAb (1 μg ml −1 , clone S5a-18, Enzo Life Sciences) or with an antibody directed against β-actin (1 μg ml −1 , Abcam). Knockdown of hRpn10 was verified with real-time RT–PCR on a Applied Biosystems 7900-HT Fast Real-Time PCR Cycler using the QuantiTect SYBR Green PCR kit (Qiagen) with specific Primers for hRpn10 (QuantiTect Primer Assay Hs_PSMD4_1_SG, Qiagen) and normalized to the expression of GAPDH. Yeast two-hybrid analysis The cDNAs encoding human FAT10 and NUB1L were cloned into the plasmid pGADT7 (Clontech) and were used as bait to screen all subunits of the human 19S RP. The cDNA of each individual human 19S RP subunits cloned into the pGBD vector (Clontech) [45] was generously provided by Robert E. Cohen (Colorado State University); Rpn13 (ref. 4 ) was also included in this test (a kind gift from Koraljka Husnjak, Frankfurt University). The bait construct was transformed into the yeast strain AH109 by standard LiCl transformation [46] and tested for self-activation by X-gal filter assay on selection plates lacking either leucine (for FAT10 and NUB1L) or tryptophan (for RP subunits). For the interaction analysis, FAT10 or NUB1L was co-transformed with the prey constructs encoding the different RP subunits. The co-transformants were grown on selection plates in the presence of 1 mM 3-AT at 30 °C. After incubation for 4 days, the colonies were replicated on Whatman filter paper, frozen in liquid nitrogen, soaked in PBS containing X-gal (100 μg ml −1 ) and incubated at room temperature. For the positive control, pLexA–FAT10 (ref. 23 ) was co-transformed with pGADT7–NUB1L in the NMY51 yeast strain. Multiple protein sequence alignment The amino-acid sequence of the VWA domain of hRpn10 of the 26S proteasome from different organisms were obtained from Conserved Domains Database ( http://www.ncbi.nlm.nih.gov/cdd ) and were aligned and formatted using Jalview [47] and ALINE [48] . The percent identity was calculated using Jalview. The alignments for N- and C-terminal hFAT10 with human ubiquitin were performed using CLUSTAL W ( http://www.ebi.ac.uk/Tools/msa/clustalw2/ ) and formatted using ALINE. How to cite this article: Rani, N. et al . FAT10 and NUB1L bind to the VWA domain of Rpn10 and Rpn1 to enable proteasome-mediated proteolysis. Nat. Commun. 3:749 doi: 10.1038/ncomms1752 (2012).